Gapless spin liquid of an organic triangular compound evidenced by thermodynamic measurements In frustrated magnetic systems, long-range ordering is forbidden and degeneracy of energy states persists, even at extremely low temperatures. Under certain conditions, these systems form an exotic quantum spin-liquid ground state, in which strongly correlated spins fluctuate in the spin lattices. Here we investigate the thermodynamic properties of an anion radical spin liquid of EtMe 3 Sb[Pd(dmit) 2 ] 2 , where dmit represents 1,3-dithiole-2-thione-4,5-dithiolate. This compound is an organic dimer-based Mott insulator with a two-dimensional triangular lattice structure. We present distinct evidence for the formation of a gapless spin liquid by examining the T -linear heat capacity coefficient, γ , in the low-temperature heat capacity. Using comparative analyses with κ-(BEDT-TTF) 2 Cu 2 (CN) 3 , a generalized picture of the new spin liquid in dimer-based organic systems is discussed. We also report anomalous enhancement of γ , produced by a kind of criticality inherent to the Pd(dmit) 2 phase diagram. The formation of a spin-liquid ground state in frustrated systems is a macroscopic manifestation of quantum phenomena associated with spin degrees of freedom. Numerous studies have investigated the nature of this fluctuating spin state at low energies [1] , [2] , [3] , [4] . Theoretical studies predict new possibilities for the ground state, namely, the long-range resonating valence bond (RVB) state, which is expressed by numerous singlet bonds resonating in the lattice [4] and other spin liquids with small-gap or gapless character in their low-energy excitations [1] , [2] , [3] . Recent advances in material syntheses and characterization techniques have resulted in various new spin liquids being produced. Two-dimensional triangular lattice compounds such as Cs 2 CuCl 4 ( S -1/2) [5] , NiGa 2 S 4 ( S -1) [6] and κ-(BEDT-TTF) 2 Cu 2 (CN) 3 ( S -1/2) [7] and Kagomé lattices of SrCr 9p Ga 12-9p O 19 ( S -3/2) [8] , volborthite ( S -1/2) [9] , herbertsmithite ( S -1/2) [10] and vesigniete ( S -1/2) [11] have stimulated extensive research. More recently, a spin-liquid state in a hyper-Kagomé lattice compound of Na 4 Ir 3 O 8 ( S -1/2) [12] was observed, enabling frustration physics in a 3D system to be investigated. Fundamental studies to understand the intrinsic nature of spin liquids and their related physical properties are advancing rapidly [13] . Among these spin-liquid materials, an organic compound of κ-(BEDT-TTF) 2 Cu 2 (CN) 3 offer unique insights into frustration physics. It is a dimer-based molecular Mott insulator with a two-dimensional structure. The electronic properties are dominated by strong magnetic interactions, | J |/ k B , larger than 200 K [7] . In this compound, spin-liquid nature has been observed by 13 C-NMR [7] , heat capacity [14] and thermal transport [15] measurements. Although the gapless feature of the low-energy excitations is reported by the heat capacity measurement [14] , thermal transport result implies a possibility of a tiny gap opening with an order of 0.5 K [15] . A possible relation with the superconductivity of conductive π-electrons and coupling with charge degrees of freedom in the dimer unit [16] are stimulating extensive interest in frustration problems and electron correlations. Recently, an anion radial compound of EtMe 3 Sb[Pd(dmit) 2 ] 2 has been reported as another candidate of organic quantum spin-liquid material by magnetic susceptibility [17] , 13 C-NMR [18] , [19] and thermal conductivity [20] measurements. EtMe 3 Sb[Pd(dmit) 2 ] 2 consists of an anion of an acceptor molecule Pd(dmit) 2 and a countercation EtMe 3 Sb + . Dimerized [Pd(dmit) 2 ] 2 − anions form a segregated stacking structure in a crystal lattice with space group C 2/ c and a quasi-two-dimensional π-electron system is established in it [21] . 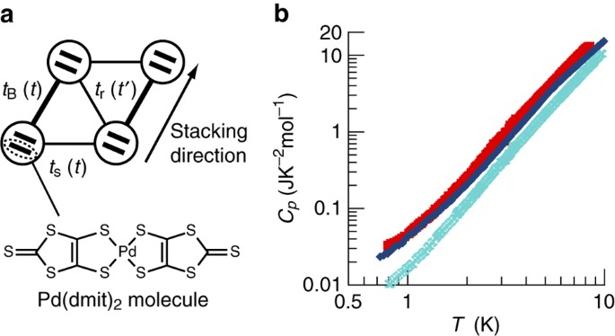Figure 1: Temperature dependences of heat capacities of EtMe3Sb[Pd(dmit)2]2and its related salts. (a) A schematic illustration of the molecular arrangement in the acceptor plane of EtMe3Sb[Pd(dmit)2]2(upper) and molecular structure of Pd(dmit)2(lower). The longer axis of the molecule is arranged perpendicular to the plane. Pd(dmit)2molecules form a dimerized structure, which is indicated by the circle. The dimers form a triangular lattice structure. The definition of three transfer integrals between neighbouring dimers (tB,tr,ts) of Pd(dmit)2systems is shown in the upper figure. The magnitude of these transfers is (tr=)t′/t(=ts≈tB) and ift′/t=1, a regular triangular system is established. The stacking direction of Pd(dmit)2molecules is shown by the arrow. (b) The data of EtMe3Sb[Pd(dmit)2]2(red squares), EtMe3P[Pd(dmit)2]2(P21/m: aqua blue crosses) and κ-(BEDT-TTF)2Cu2(CN)3(blue diamonds) are plotted on a logarithmic scale. The heat capacities of spin-liquid compounds EtMe3Sb[Pd(dmit)2] and κ-(BEDT-TTF)2Cu2(CN)3are larger than those of EtMe3P[Pd(dmit)2]2with ordered ground state due to the spin entropy remains at low temperatures in the former two compounds. The realization of the spin-liquid state is suggested in EtMe3Sb[Pd(dmit)2]2. Figure 1a shows the molecular structure of Pd(dmit) 2 and crystal packing in the 2D plane. As the energy gap between the highest occupied molecular orbital (HOMO) and the lowest unoccupied molecular orbital (LUMO) is small, an electron spin localized on each dimer originates from the antibonding HOMOs [22] . The d -orbital of the Pd ion makes a negligible contribution to the HOMO and thus does not contribute to the spin density. By changing the central pnictogen atom and the numbers of methyl (Me) and ethyl (Et) groups in countercations, the ratio of the transfer integrals between the dimers ( t r =) t ′/ t (= t s ≈ t B ) shown in the inset of Figure 1a can be tuned from the antiferromagnetic (AF) region to the charge-ordered (CO) region in the phase diagram [23] . Tight-binding calculations based on the crystallographic data at room temperature suggest that the compound of EtMe 3 Sb[Pd(dmit) 2 ] 2 is located at t ′ /t =0.92, which implies that a nearly ideal triangle structure is realized [18] , [24] . This compound is similar to κ-(BEDT-TTF) 2 Cu 2 (CN) 3 ; they are Mott insulators with a layered structure consisting of a triangular lattice of dimers. The remarkable structural feature of EtMe 3 Sb[Pd(dmit) 2 ] 2 is that it has a stacking direction of acceptor molecules, shown in Figure 1a , which is a characteristic factor in discussing the Pd(dmit) 2 compounds. Figure 1: Temperature dependences of heat capacities of EtMe 3 Sb[Pd(dmit) 2 ] 2 and its related salts. ( a ) A schematic illustration of the molecular arrangement in the acceptor plane of EtMe 3 Sb[Pd(dmit) 2 ] 2 (upper) and molecular structure of Pd(dmit) 2 (lower). The longer axis of the molecule is arranged perpendicular to the plane. Pd(dmit) 2 molecules form a dimerized structure, which is indicated by the circle. The dimers form a triangular lattice structure. The definition of three transfer integrals between neighbouring dimers ( t B , t r , t s ) of Pd(dmit) 2 systems is shown in the upper figure. The magnitude of these transfers is ( t r =) t ′/ t (= t s ≈ t B ) and if t ′/ t =1, a regular triangular system is established. The stacking direction of Pd(dmit) 2 molecules is shown by the arrow. ( b ) The data of EtMe 3 Sb[Pd(dmit) 2 ] 2 (red squares), EtMe 3 P[Pd(dmit) 2 ] 2 (P2 1 /m: aqua blue crosses) and κ-(BEDT-TTF) 2 Cu 2 (CN) 3 (blue diamonds) are plotted on a logarithmic scale. The heat capacities of spin-liquid compounds EtMe 3 Sb[Pd(dmit) 2 ] and κ-(BEDT-TTF) 2 Cu 2 (CN) 3 are larger than those of EtMe 3 P[Pd(dmit) 2 ] 2 with ordered ground state due to the spin entropy remains at low temperatures in the former two compounds. The realization of the spin-liquid state is suggested in EtMe 3 Sb[Pd(dmit) 2 ] 2 . Full size image In this study, we report the low-temperature thermodynamic nature of EtMe 3 Sb[Pd(dmit) 2 ] 2 focusing on the low-energy excitations from the ground state. From the thermodynamic data, we assert that the ground state is a gapless spin liquid characterized by the existence of a distinct T -linear heat capacity term. Comparative discussions on the Wilson ratio, R W , and a hump-like structure with κ-(BEDT-TTF) 2 Cu 2 (CN) 3 reveal that the spin liquids of organic compounds have similar characters. Our low-temperature heat capacity data of deuterated EtMe 3 Sb[Pd(dmit) 2 ] 2 imply a possible enhancement of heat capacity around the quantum critical region of the AF and spin liquid in the phase diagram. Heat capacities of EtMe 3 Sb[Pd(dmit) 2 ] 2 and its analogues The temperature dependence of the heat capacity of EtMe 3 Sb[Pd(dmit) 2 ] 2 obtained by measuring several crystals is shown in Figure 1b . The heat capacities are plotted on a logarithmic scale against temperature. Data for κ-(BEDT-TTF) 2 Cu 2 (CN) 3 [14] are also displayed in the figure, which show qualitatively similar temperature dependence. The heat capacity of EtMe 3 Sb[Pd(dmit) 2 ] 2 has no sharp peak structure. This result indicates absence of long-range orderings over the entire measured temperature range. Figure 1b also displays data for EtMe 3 P[Pd(dmit) 2 ] 2 ( P 2 1 / m ), which has a non-magnetic ground state with valence bond solid (VBS) type ordering at 25 K [23] , [25] . The heat capacity values, for example, 42.8 mJ K −1 mol −1 at 1 K and 115 mJ K −1 mol −1 at 4 K of EtMe 3 Sb[Pd(dmit) 2 ] 2 , which are relatively higher than those for EtMe 3 P[Pd(dmit) 2 ] 2 , indicate that magnetic entropy survives at low temperature owing to fluctuations of correlated spins. The absence of thermal anomalies is consistent with the magnetic susceptibility measurement down to 5 K performed by Tamura and Kato [17] and the 13 C-NMR spectrum down to 19.4 mK measured by Itou et al . 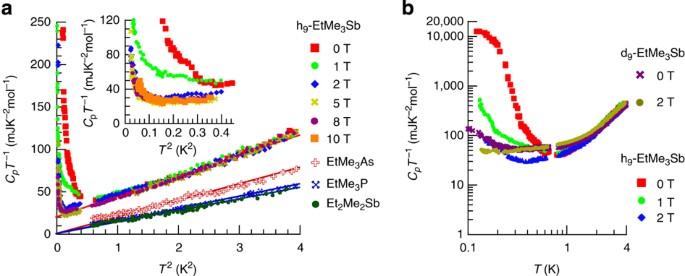Figure 2: Low-temperature heat capacities of EtMe3Sb[Pd(dmit)2]2. (a)CpT−1versusT2plot of EtMe3Sb[Pd(dmit)2]2(h9-EtMe3Sb) below 2 K obtained under 0 T (red squares), 1 T (green filled circles), 2 T (blue diamonds), 5 T (ocher crosses) and 8 T (purple filled circles). This figure contains the data of related Pd(dmit)2salts of EtMe3As[Pd(dmit)2]2(EtMe3As red pluses), EtMe3P[Pd(dmit)2]2(EtMe3P blue crosses) and Et2Me2Sb[Pd(dmit)2]2(Et2Me2Sb green filled circles), which have ordered ground states for comparison. The fitting lines obtained by using the data of 0 T of each salt are shown by the same colours with the data. The existence of aT-linear contribution even in the insulating state of EtMe3Sb[Pd(dmit)2]2is observed. A large upturn below 1 K that masks the information of the electron spins is probably attributable to the rotational tunnelling of Me groups. The inset figure showsCpT−1versusT2plot of EtMe3Sb[Pd(dmit)2]2data below 0.7 K, where a large upturn with magnetic field dependence appears. The data obtained under 0 T (red squares), 1 T (green filled circles), 2 T (blue diamonds), 5 T (ocher crosses), 8 T (purple filled circles) and 10 T (orange squares) are plotted. (b) The overall behaviour ofCpT−1below 4 K of EtMe3Sb[Pd(dmit)2]2(h9-EtMe3Sb) and its deuterated compound of d9-EtMe3Sb[Pd(dmit)2]2(d9-EtMe3Sb) in a logarithmic plot. The data under 0 T (red squares), 1 T (green filled circles) and 2 T (blue diamonds) of EtMe3Sb[Pd(dmit)2]2is shown by the same symbols as in (a). The data obtained under 0 T (purple crosses) and 2 T (ocher filled circles) of d9-EtMe3Sb[Pd(dmit)2]2are compared in the same plot. The upturn has been reduced down to about few percent by deuteration. The origin of the upturn is extrinsic for the discussion of electronic spins and is attributed to the existence of rotational tunnelling levels of Me groups in the cation. [18] , [19] To elucidate the detailed characteristics of low-energy excitations from the ground state, data in the low-temperature region are plotted as C p T −1 vs T 2 in Figure 2a . Fitting the 0-T data between 0.9 and 2.0 K for EtMe 3 Sb[Pd(dmit) 2 ] 2 using the formula C p T −1 = γ + βT 2 gives γ =19.9 mJ K −2 mol −1 and β =24.1 mJ K −4 mol −1 . The finite electronic heat capacity coefficient γ in a triangular S -1/2 spin system suggests that gapless excitations occur from a liquid-like ground state, similar to the case of κ-(BEDT-TTF) 2 Cu 2 (CN) 3 [14] . As Figure 2a shows, γ is not seriously affected by magnetic fields up to 8 T. This excludes the possibility that paramagnetic impurity spins are the origin of the γ term. The measurement was also performed for over 50 pieces of microcrystals, and the temperature and magnetic field dependences obtained were almost the same as those in Figure 2a . Thus, the large heat capacity at low temperatures is attributed to the intrinsic properties of this material. Figure 2: Low-temperature heat capacities of EtMe 3 Sb[Pd(dmit) 2 ] 2 . ( a ) C p T −1 versus T 2 plot of EtMe 3 Sb[Pd(dmit) 2 ] 2 (h 9 -EtMe 3 Sb) below 2 K obtained under 0 T (red squares), 1 T (green filled circles), 2 T (blue diamonds), 5 T (ocher crosses) and 8 T (purple filled circles). This figure contains the data of related Pd(dmit) 2 salts of EtMe 3 As[Pd(dmit) 2 ] 2 (EtMe 3 As red pluses), EtMe 3 P[Pd(dmit) 2 ] 2 (EtMe 3 P blue crosses) and Et 2 Me 2 Sb[Pd(dmit) 2 ] 2 (Et 2 Me 2 Sb green filled circles), which have ordered ground states for comparison. The fitting lines obtained by using the data of 0 T of each salt are shown by the same colours with the data. The existence of a T -linear contribution even in the insulating state of EtMe 3 Sb[Pd(dmit) 2 ] 2 is observed. A large upturn below 1 K that masks the information of the electron spins is probably attributable to the rotational tunnelling of Me groups. The inset figure shows C p T −1 versus T 2 plot of EtMe 3 Sb[Pd(dmit) 2 ] 2 data below 0.7 K, where a large upturn with magnetic field dependence appears. The data obtained under 0 T (red squares), 1 T (green filled circles), 2 T (blue diamonds), 5 T (ocher crosses), 8 T (purple filled circles) and 10 T (orange squares) are plotted. ( b ) The overall behaviour of C p T −1 below 4 K of EtMe 3 Sb[Pd(dmit) 2 ] 2 (h 9 -EtMe 3 Sb) and its deuterated compound of d 9 -EtMe 3 Sb[Pd(dmit) 2 ] 2 (d 9 -EtMe 3 Sb) in a logarithmic plot. The data under 0 T (red squares), 1 T (green filled circles) and 2 T (blue diamonds) of EtMe 3 Sb[Pd(dmit) 2 ] 2 is shown by the same symbols as in (a). The data obtained under 0 T (purple crosses) and 2 T (ocher filled circles) of d 9 -EtMe 3 Sb[Pd(dmit) 2 ] 2 are compared in the same plot. The upturn has been reduced down to about few percent by deuteration. The origin of the upturn is extrinsic for the discussion of electronic spins and is attributed to the existence of rotational tunnelling levels of Me groups in the cation. Full size image To disclose peculiarity in the thermodynamic properties due to spin frustration, Figure 2a also shows the data for two other analogous compounds EtMe 3 As[Pd(dmit) 2 ] 2 and Et 2 Me 2 Sb[Pd(dmit) 2 ] 2 , together with the data for EtMe 3 P[Pd(dmit) 2 ] 2 . These salts have ordered ground states as are assorted by their transfer energy ratios t ′/ t . EtMe 3 P[Pd(dmit) 2 ] 2 has a nonmagnetic VBS state below 25 K [25] , whereas EtMe 3 As[Pd(dmit) 2 ] 2 has an antiferromagnetic long-range ordering at 23 K [26] . Et 2 Me 2 Sb[Pd(dmit) 2 ] 2 undergoes a drastic first-order transition accompanied by CO at 70 K [27] . From the figure, it is evident that these salts with ordered ground states have lower heat capacities than EtMe 3 Sb[Pd(dmit) 2 ] 2 . Linear extrapolation of the data to T =0 gives a vanishing γ term in the heat capacity. This fact demonstrates that the T -linear contribution is observed only in the spin-liquid system. Heat capacity of EtMe 3 Sb[Pd(dmit) 2 ] 2 below 1 K As frustrated spin systems may undergo unexpected phase changes in the low-energy region due to various kinds of many-body effects, thermodynamic measurements should be performed at temperatures as low as possible. In Figure 2a , we also show heat capacity data obtained in the dilution temperature region in the C p T −1 vs T 2 plot. These data are displayed in the inset of Figure 2a , wherein a low-temperature region is expanded in the same plot. Unexpectedly, a large upturn below 1 K masks information about the electron spins. The magnetic fields tend to reduce this upturn, which is an unusual behaviour as a simple Schottky-type heat capacity due to nuclear spins. Figure 2b is a logarithmic plot that shows the overall behaviour of C p T −1 below 4 K. The most plausible explanation for this upturn is rotational motion of methyl (Me) groups in the cation layer. The Me groups have a hindered rotation due to quantum tunnelling in the threefold symmetry potential ( C 3 ) at low temperatures. The energy levels of the quantum tunnelling states are expressed by irreducible representation of A , E, and there exists a small energy splitting expressed by Δ between them. These levels are coupled with nuclear spin states of three protons in the Me group. If the proton spins are in equilibrium condition, the total nuclear spins for A and E states should be I =3/2 and I =1/2, respectively. The energy splitting (Δ) is usually very small, in the order of 10 0−2 μeV, and therefore produces an increase of heat capacity corresponding to the high-temperature tail of the Schottky anomaly below 1 K, as is studied by Sorai et al . in some metal complexes containing Me groups [28] . The upturn observed in EtMe 3 Sb[Pd(dmit) 2 ] 2 is considered to have the same origin. Application of a magnetic field may cause a hyperfine splitting of the nuclear spins and it consequently creates magnetic-field dependence in C p . However, spin inversion of protons in such organic salts has a rather long spin-lattice relaxation time, in the order of 10 1–3 s, so that it cannot be detected accurately by thermal relaxation calorimetry technique, in which we usually analyse temperature relaxation behaviours in the similar time scale. The unusual magnetic field dependence of this Schottky anomaly under magnetic fields observed in this compound is probably related to the behaviours of nuclear spin levels and to the long time constant of proton spin inversion. This remains speculative because, to the best of our knowledge, the detailed magnetic-field dependence of the heat capacity has not been investigated experimentally. However, the unexpectedly large heat capacity, which is comparable to the electron spin entropy in this limited temperature region, suggests that it should be considered separately from the electronic system. The estimation of γ using the dilution temperature data does not reveal any change, which implies that the T -linear term with γ =19.9 mJ K −2 mol −1 is intrinsic for this material. The C p T −1 vs T 2 plots in Figure 2a for EtMe 3 Sb[Pd(dmit) 2 ] 2 under relatively strong magnetic fields of 8 T in the 3 He region and up to 10 T in the dilution temperature region do not reveal any significant change in the γ term. A T -linear term of the low-temperature heat capacity with a similar magnitude was reported for κ-(BEDT-TTF) 2 Cu 2 (CN) 3 as evidence of gapless excitations from the spin-liquid ground state [14] . The subsequent thermal conductivity measurement suggested a possibility of a tiny gap of about Δ=0.016 J / k B [15] , the origin of which is still an open question. The gapless thermal excitations observed in the heat capacity of the present salt are consistent with the thermal conductivity data obtained by Yamashita et al . [20] Samples of κ-(BEDT-TTF) 2 Cu 2 (CN) 3 may sometimes contain impurities due to Cu 2+ and disorders depending on a difference of crystal growth conditions as is suggested in the previous works [14] , [29] , [30] . However, EtMe 3 Sb[Pd(dmit) 2 ] 2 samples used in the present study seem to be of better quality, judging from the smaller sample dependences and the absence of paramagnetic impurities behaviour in the magnetic field dependence. The consistency of the heat capacity and the thermal transport results ensures that the spin-liquid state realized in this compound has a gapless character. Deuteration effects on thermodynamic properties In order to confirm that the upturn is originated from the rotational tunnelling, we also measured the heat capacity of a d 9 -EtMe 3 Sb[Pd(dmit) 2 ] 2 compound in which three Me groups in the cation had been deuterated during synthesis. As is shown in Figure 2b , the upturn was reduced down to a few percent due to the increased mass of Me groups. The residual upturn is inferred to be a trace of non-deuterated Me groups and Et groups remaining in the cations. The magnetic field dependence of the residual upturn of the deuterated compound shown in Figure 2b is the same as that of the pristine compound, which also ensures that this term is arisen by rotational tunnelling. Interestingly, we found that the deuterated compound in Figure 2b has a larger C p T −1 in the higher-temperature region up to about 2 K, which should be considered separately from the contribution of Me groups. 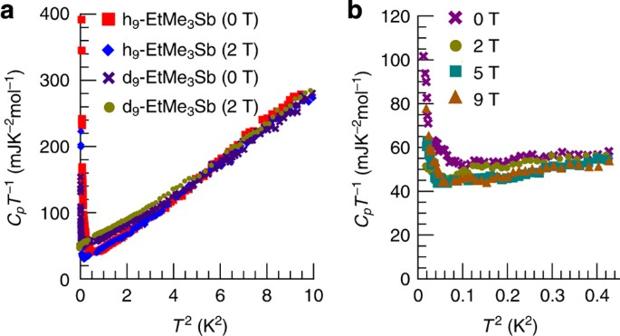Figure 3: Comparison of electronic heat capacity coefficientγbetween EtMe3Sb[Pd(dmit)2]2and d9-EtMe3Sb[Pd(dmit)2]2. (a) Low-temperature heat capacities of h9-EtMe3Sb[Pd(dmit)2]2(h9-EtMe3Sb; 0 T red squares, 2 T blue diamonds) and d9-EtMe3Sb[Pd(dmit)2]2(d9-EtMe3Sb; 0 T purple pluses, 2 T ocher filled circles) below 3.1 K. Upward deviation of heat capacities of d9-EtMe3Sb[Pd(dmit)2]2is observed below 2 K. The enhancement of the electronic heat capacity of d9-EtMe3Sb[Pd(dmit)2]2is realized in this temperature region. (b) Low-temperature heat capacities of d9-EtMe3Sb[Pd(dmit)2]20 T (purple crosses), 2 T (ocher filled circles), 5 T (aqua blue squares) and 9 T (orange triangles) below 0.65 K plotted inCpT−1versusT2. The enhancedT-linear contribution in heat capacity does not have drastic magnetic field dependence. Comparison of heat capacity data of the deuterated compound and pristine compound is shown in a wider temperature scale in Figure 3a . The temperature dependence of C p T −1 of the deuterated compound coincides well with that of the pristine compound above 2 K; however, below this temperature, it deviates upward with decreasing temperature. This deviation is gradual and insensitive to the external magnetic field of 2 T, but extrapolation down to T =0 gives a γ of about 40 mJ K −2 mol −1 , which is nearly twice as large as that of the pristine compound. Figure 3b shows the data in the lower-temperature region under magnetic fields. The enhancement of the γ is retained and is observed under magnetic fields up to 9 T. Figure 3: Comparison of electronic heat capacity coefficient γ between EtMe 3 Sb[Pd(dmit) 2 ] 2 and d 9 -EtMe 3 Sb[Pd(dmit) 2 ] 2 . ( a ) Low-temperature heat capacities of h 9 -EtMe 3 Sb[Pd(dmit) 2 ] 2 (h 9 -EtMe 3 Sb; 0 T red squares, 2 T blue diamonds) and d 9 -EtMe 3 Sb[Pd(dmit) 2 ] 2 (d 9 -EtMe 3 Sb; 0 T purple pluses, 2 T ocher filled circles) below 3.1 K. Upward deviation of heat capacities of d 9 -EtMe 3 Sb[Pd(dmit) 2 ] 2 is observed below 2 K. The enhancement of the electronic heat capacity of d 9 -EtMe 3 Sb[Pd(dmit) 2 ] 2 is realized in this temperature region. ( b ) Low-temperature heat capacities of d 9 -EtMe 3 Sb[Pd(dmit) 2 ] 2 0 T (purple crosses), 2 T (ocher filled circles), 5 T (aqua blue squares) and 9 T (orange triangles) below 0.65 K plotted in C p T −1 versus T 2 . The enhanced T -linear contribution in heat capacity does not have drastic magnetic field dependence. Full size image Broad hump structure in heat capacity In the case of κ-(BEDT-TTF) 2 Cu 2 (CN) 3 , the low-temperature quantum liquid state is realized below a crossover temperature of 5.7 K, at which the heat capacity has a broad hump structure [14] . Recent thermal expansion measurements by Manna et al . [31] indicate a clear anomaly at this temperature. Abdel-Jawad et al . [16] have suggested that the unusual dielectric properties at higher temperatures are related to charge disproportionation in dimers. 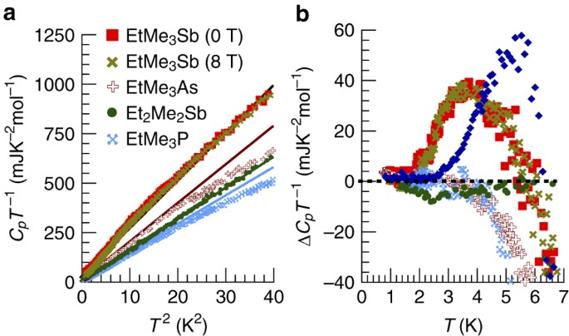Figure 4: Analyses of temperature dependences of the heat capacity of Pd(dmit)2salts. (a)CpT−1versusT2plots of the heat capacity of EtMe3Sb[Pd(dmit)2]2(EtMe3Sb; 0 T red squares, 8 T ocher crosses), EtMe3As[Pd(dmit)2]2(EtMe3As; 0 T purple pluses), Et2Me2Sb[Pd(dmit)2]2(Et2Me2Sb; 0 T green filled circles) and EtMe3P[Pd(dmit)2]2(EtMe3P; 0 T aqua blue crosses). The lines shown in the figure areβT3terms determined by the low-temperature data below 2.0 K. Around 3–4 K, a broad hump structure is observed only in EtMe3Sb[Pd(dmit)2]2. The data obtained under 8 T of EtMe3Sb[Pd(dmit)2]2also show the hump structure. (b) The temperature dependences of ΔCp=Cp−βT3defined as a difference of the heat capacity data from the βT3for each compound in (a) are shown in ΔCpT−1vsTplot. The symbols of the data are the same as those shown in (a). The data clearly indicate that the broad hump structure exists only in EtMe3Sb[Pd(dmit)2]2in the Pd(dmit)2system. The result of similar analysis for κ-(BEDT-TTF)2Cu2(CN)3(blue diamonds) is also presented in the figure. As shown in Figure 4a, a similar broad hump structure is observed in the C p T −1 vs T 2 curve of EtMe 3 Sb[Pd(dmit) 2 ] 2 . Comparison with the data for EtMe 3 P[Pd(dmit) 2 ] 2 , EtMe 3 As[Pd(dmit) 2 ] 2 and Et 2 Me 2 Sb[Pd(dmit) 2 ] 2 in Figure 4a reveals the hump structure in the EtMe 3 Sb[Pd(dmit) 2 ] 2 data. The lines in Figure 4a represent the βT 3 term determined from the low-temperature data below 2.0 K for these compounds. The β value is 24.1 mJ K −4 mol −1 for EtMe 3 Sb[Pd(dmit) 2 ] 2 , 14.3 mJ K −4 mol −1 for EtMe 3 P[Pd(dmit) 2 ] 2 , 19.5 mJ K −4 mol −1 for EtMe 3 As[Pd(dmit) 2 ] 2 and 13.2 mJ K −4 mol −1 for Et 2 Me 2 Sb[Pd(dmit) 2 ] 2 . Deviations of the experimental data of C p from βT 3 are determined using the formula Δ C p = C p − βT 3 , and Δ C p T −1 values of these compounds are plotted as a function of temperature in Figure 4b . The data of EtMe 3 Sb[Pd(dmit) 2 ] 2 clearly reveal the broad hump structure. Figure 4b also shows additional heat capacity due to the hump in the κ-(BEDT-TTF) 2 Cu 2 (CN) 3 [14] obtained by similar analysis. The hump temperature and the magnitude of the Δ C p T −1 peak of EtMe 3 Sb[Pd(dmit) 2 ] 2 are, respectively, about 3.7 K and 35 mJ K −1 mol −1 , whereas they are, respectively, 5.7 K and 60 mJ K −2 mol −1 for κ-(BEDT-TTF) 2 Cu 2 (CN) 3 . As the lattice heat capacities of organic salts do not obey the simple βT 3 term around the hump temperature of κ-(BEDT-TTF) 2 Cu 2 (CN) 3 , Δ C p T −1 does not reflect the correct magnetic heat capacity in this compound. The lattice heat capacity has been more accurately estimated in our previous work using the lattice heat capacities of similar κ-(BEDT-TTF) 2 X compounds, and the excess entropy of the hump was estimated to be 700–1,000 mJ K −1 mol −1 (ref. 14 ). The excess entropy related to the hump in the EtMe 3 Sb[Pd(dmit) 2 ] 2 data is approximately evaluated as 70–100 mJ K −1 mol −1 , which is 7–14% of that of κ-(BEDT-TTF) 2 Cu 2 (CN) 3 . The hump temperatures of both salts seem to correspond to temperatures at which a small dip-like structure appears in the temperature dependences of T 1 −1 obtained by Itou et al . for EtMe 3 Sb[Pd(dmit) 2 ] 2 (ref. 18 ) and by Shimizu et al . for κ-(BEDT-TTF) 2 Cu 2 (CN) 3 (ref. 7 ). Figure 4b also reveals that this hump structure of EtMe 3 Sb[Pd(dmit) 2 ] 2 does not have a magnetic field dependence up to 8 T. Figure 4: Analyses of temperature dependences of the heat capacity of Pd(dmit) 2 salts. ( a ) C p T −1 versus T 2 plots of the heat capacity of EtMe 3 Sb[Pd(dmit) 2 ] 2 (EtMe 3 Sb; 0 T red squares, 8 T ocher crosses), EtMe 3 As[Pd(dmit) 2 ] 2 (EtMe 3 As; 0 T purple pluses), Et 2 Me 2 Sb[Pd(dmit) 2 ] 2 (Et 2 Me 2 Sb; 0 T green filled circles) and EtMe 3 P[Pd(dmit) 2 ] 2 (EtMe 3 P; 0 T aqua blue crosses). The lines shown in the figure are βT 3 terms determined by the low-temperature data below 2.0 K. Around 3–4 K, a broad hump structure is observed only in EtMe 3 Sb[Pd(dmit) 2 ] 2 . The data obtained under 8 T of EtMe 3 Sb[Pd(dmit) 2 ] 2 also show the hump structure. ( b ) The temperature dependences of Δ C p = C p −β T 3 defined as a difference of the heat capacity data from the β T 3 for each compound in ( a ) are shown in Δ C p T −1 vs T plot. The symbols of the data are the same as those shown in ( a ). The data clearly indicate that the broad hump structure exists only in EtMe 3 Sb[Pd(dmit) 2 ] 2 in the Pd(dmit) 2 system. The result of similar analysis for κ-(BEDT-TTF) 2 Cu 2 (CN) 3 (blue diamonds) is also presented in the figure. Full size image The gapless excitations observed by the heat capacity measurements can be discussed qualitatively by assuming finite density of states in spin excitations. The temperature dependence of the magnetic susceptibility of EtMe 3 Sb[Pd(dmit) 2 ] 2 has a broad peak around 60 K, which corresponds to a two-dimensional Heisenberg model of a triangular lattice with a magnetic interaction – J/k B =220–250 K. Extrapolating the temperature dependence of the spin susceptibility down to T =0 gives a residual magnetic susceptibility of χ (0). For EtMe 3 Sb[Pd(dmit) 2 ] 2 , χ (0) is estimated to be 4.4×10 −4 emu mol −1 from the data obtained by Tamura et al . [17] Using the value of γ determined in the present study, the Wilson ratio, R W , is evaluated to be 1.09. In the case of κ-(BEDT-TTF) 2 Cu 2 (CN) 3 , χ (0) is 2.9×10 −4 emu mol −1 and γ is determined as 12.6 mJ K −2 mol −1 from the data in the dilution temperature region [7] , [14] , which gives an R W of 1.13. These very similar values of R W imply a proper scaling of χ (0) and γ exists in the organic spin-liquid state. A Wilson ratio in the order of unity is typical for a Fermi liquid with nearly free electrons. 13 C-NMR measurements by Itou et al . suggest a transition around 1 K and nodal type excitations in the spin-lattice relaxation time similar to those for d -wave superconductivity [32] . At present, it is difficult to reconcile 13 C-NMR data with the thermodynamic data, but this discrepancy may give a further problem related to the dynamics due to the strong correlations in spin liquids. Although the liquid-like states of the two organic salts exhibit similar thermodynamic properties, their phase diagrams surrounding the spin-liquid phase are different. Here, we discuss the difference in the γ terms of pristine and deuterated samples of EtMe 3 Sb[Pd(dmit) 2 ] 2 in terms of the electron-phase diagram. 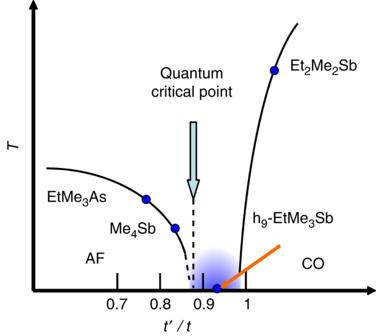Figure 5: A schematic view of electronic phase diagram of the Pd(dmit)2system. The electronic properties of Pd(dmit)2system are dominated byt/t′ ratio. The spin-liquid phase is located in the narrow region between antiferromagnetic (AF) and charge order (CO) phases. The positions of EtMe3Sb[Pd(dmit)2]2(h9-EtMe3Sb), EtMe3As[Pd(dmit)2]2(EtMe3As), Me4Sb[Pd(dmit)2]2(Me4Sb) and Et2Me2Sb[Pd(dmit)2]2(Et2Me2Sb) are indicated in the figure. Figure 5 shows a schematic electronic phase diagram of the Pd(dmit) 2 system, which reveals that the spin-liquid phase occurs in a narrow region. The AF phase and CO phase are both suppressed around the spin-liquid phase [23] . The AF phase is suppressed due to the increase in the frustration effects denoted by t ′/ t. The point at which T N is reduced to 0 is defined as a quantum critical point between spin-solid and liquid states. As mentioned above, the pristine EtMe 3 Sb[Pd(dmit) 2 ] 2 is located in the spin-liquid state with t ′/ t =0.92. Deuteration of the Me groups slightly reduces the cation size and moves the electronic state from the spin-liquid region toward the AF region, as Me 4 Sb[Pd(dmit) 2 ] 2 , which has a smaller cation, is located in the AF phase [17] . A possible explanation of the enhancement in the γ term is that the deuterated compound is located very close to the critical point, which causes a critical divergence in its thermodynamic properties. In heavy-electron systems produced by strong correlations of f -electrons in Ce and U compounds, anomalous divergence of C p T −1 expressed by the −log T term is known as a non-Fermi liquid behaviour at the quantum critical point [33] , where the AF phase is suppressed to T N =0 and an anomalous Fermi liquid phase appears. A similar kind of criticality might be expected in the critical region of a spin-liquid phase. Precise tuning of electronic properties by chemical pressures generated by partial substitution of deuterons in molecules has been achieved in the (DMe-DCNQI) 2 Cu system [34] ; this should also be possible by controlling the cations in Pd(dmit) 2 systems. Another possible explanation of this γ enhancement is related to the nodal structure produced in the low-energy excitations in the gap. If a finite density of states at zero energy was detected as the γ term in thermodynamic experiments, like in d -wave superconductivity, as is suggested by a theoretical study by Grover et al . [35] and the NMR experiments [32] , it might be sensitive to slight changes in the chemical pressure in the spin-liquid phase. A further possible explanation is a change in the disorder potential produced by the low symmetries of cations. Although these possibilities remain speculative, the low-energy excitations in this organic spin-liquid state contain important implications for electron correlation problems peculiar to Mott-insulator triangular systems. In contrast to this complicated situation in the Pd(dmit) 2 system, the phase diagram around the spin-liquid phase of κ-(BEDT-TTF) 2 Cu 2 (CN) 3 is relatively simple and it retains a spin-liquid ground state up to 0.36 GPa as reported by Kurosaki et al . [36] Above this pressure, the spin-liquid phase undergoes a first-order transition and a superconductive phase appears [36] . The deuterated sample of κ-(d 8 ; BEDT-TTF) 2 Cu 2 (CN) 3 shows very similar thermodynamic behaviour as the hydrogenated samples, which is in fine contrast with the EtMe 3 Sb[Pd(dmit) 2 ] 2 system [29] . The presence of a quantum criticality in the spin-liquid state may have interesting implications for organic triangular compounds. Figure 5: A schematic view of electronic phase diagram of the Pd(dmit) 2 system. The electronic properties of Pd(dmit) 2 system are dominated by t/t ′ ratio. The spin-liquid phase is located in the narrow region between antiferromagnetic (AF) and charge order (CO) phases. The positions of EtMe 3 Sb[Pd(dmit) 2 ] 2 (h 9 -EtMe 3 Sb), EtMe 3 As[Pd(dmit) 2 ] 2 (EtMe 3 As), Me 4 Sb[Pd(dmit) 2 ] 2 (Me 4 Sb) and Et 2 Me 2 Sb[Pd(dmit) 2 ] 2 (Et 2 Me 2 Sb) are indicated in the figure. Full size image In conclusion, we have performed heat capacity measurements of single crystals of EtMe 3 Sb[Pd(dmit) 2 ] 2 and found that the low-temperature electronic state is a gapless spin liquid. The existence of a finite γ term in the heat capacity of EtMe 3 Sb[Pd(dmit) 2 ] 2 strongly suggests that dense gapless excitations exist in the spin-liquid state. The magnitude of γ scales to the magnetic susceptibility with a Wilson ratio of R w =1.09. The heat capacity data of EtMe 3 Sb[Pd(dmit) 2 ] 2 exhibits a small hump structure in C p T −1 . These are common features with the quantum spin liquid in κ-(BEDT-TTF) 2 Cu 2 (CN) 3 . On the other hand, deuteration of the Me groups in EtMe 3 Sb[Pd(dmit) 2 ] 2 results in anomalous enhancement of the γ term, as it is located in the critical region between AF and CO phases. Sample preparation The single-crystal samples used in this study were synthesized by air oxidation of (EtMe 3 Sb) 2 [Pd(dmit) 2 ] in acetone containing acetic acid at 5°C. The deuterated crystals were prepared by the same method using (Et(CD) 3 Sb) 2 [Pd(dmit) 2 ]. The deuterium atoms were introduced by CD 3 I (99.5%D). Heat capacity measurements Low-temperature heat capacity measurements were performed using a thermal relaxation calorimeter constructed by ourselves for measuring single crystals of molecular compounds. We used calorimetry cells that cover the temperature ranges of 0.8–10 K and 100 mK–0.6 K. Small-chip ruthenium oxide sensors with resistances of 10 and 1 kΩ at room temperature were calibrated at 0 T and under magnetic fields up to 10 T. The sample stage was connected to a heat sink by eight constantan wires, each of diameter 13 μm. The heat leak was adjusted so as to achieve an appropriate time constant for the temperature relaxation (typically 10 1–3 s) over the whole temperature range. We used several EtMe 3 Sb[Pd(dmit) 2 ] 2 single crystals that had a total weight of 377.2 μg for a 3 He system and 297.7 μg for a dilution refrigerator system. Experiments on other salts were also performed for crystals weighing about 100 μg. The crystals were attached to the stage using a suitable amount of Apiezon N grease. Background heat capacities, including that of the Apiezon N grease, were determined by independent measurements performed before mounting the samples. The absolute heat capacities were obtained by subtracting the background values from the total heat capacity. We also measured the heat capacity of a microcrystalline sample of EtMe 3 Sb[Pd(dmit) 2 ] 2 in order to check the sample dependence. How to cite this article : Yamashita, S. et al . Gapless spin liquid of an organic triangular compound evidenced by thermodynamic measurements. Nat. Commun. 2:275 doi: 10.1038/ncomms1274 (2011).